Experimental diagenesis of organo-mineral structures formed by microaerophilic Fe(II)-oxidizing bacteria Twisted stalks are organo-mineral structures produced by some microaerophilic Fe(II)-oxidizing bacteria at O 2 concentrations as low as 3 μM. The presence of these structures in rocks having experienced a diagenetic history could indicate microbial Fe(II)-oxidizing activity as well as localized abundance of oxygen at the time of sediment deposition. Here we use spectroscopy and analytical microscopy to evaluate if—and what kind of—transformations occur in twisted stalks through experimental diagenesis. Unique mineral textures appear on stalks as temperature and pressure conditions increase. Haematite and magnetite form from ferrihydrite at 170 °C–120 MPa. Yet the twisted morphology of the stalks, and the organic matrix, mainly composed of long-chain saturated aliphatic compounds, are preserved at 250 °C–140 MPa. Our results suggest that iron minerals might play a role in maintaining the structural and chemical integrity of stalks under diagenetic conditions and provide spectroscopic signatures for the search of ancient life in the rock record. Morphological signatures are usually the first evidence used to localize putative microfossils in the rock record, yet they must be associated with robust (geo)chemical and isotopic signatures to demonstrate their biogenic origin [1] , [2] . The preservation of microfossils appears best in cherts, for example, see ref. 3 , consequently most microbial fossilization experiments performed so far have consisted in evaluating the preservation of microorganisms in silica solutions at ambient conditions for various periods of time, for example, see refs 4 , 5 , 6 , 7 . Nonetheless, a few studies have revealed that the presence of Fe in solution improves the preservation of bacterial and archaeal cell walls in silica [8] , [9] . Also the formation of Fe minerals in the cell wall of the nitrate-dependent Fe(II)-oxidizing bacterium Acidovorax sp. BoFeN1 leads to the preservation of protein globules and peptidoglycan [10] . Microorganisms involved in biomineralization processes thus represent potential candidates to be preserved in the rock record [11] , [12] . Although diagenetic and metamorphic events can significantly affect the chemical and physical content of sediments, only few studies have investigated the effects of temperature ( T ) and/or pressure ( P ) on microbial cells and extracellular microbial structures. The shape of cells of Acidovorax sp. BoFeN1 completely encrusted in Fe minerals is preserved after heating for 20 h at 600 °C or for 100 h at 300 °C, although the protein content decreases with increasing temperature [12] . Calcified cells of Escherichia coli are still recognizable after heating at 600 °C for 20 h, whereas non-calcified cells are completely destroyed under the same conditions [13] . Silicified cyanobacterial sheaths and cells start to alter after 2 weeks and degrade after 4 weeks at 165 °C and 300 MPa (refs 14 , 15 ). In the present study, we chose to investigate microbial extracellular structures under diagenetic conditions, as these structures are bigger and easier to find in the rock record than microbial cells. Twisted stalks are extracellular ribbon-like organo-mineral structures produced by neutrophilic microaerophilic, freshwater and marine Fe(II)-oxidizing bacteria (FeOB) in the β-Proteobacteria and ζ-Proteobacteria phyla, respectively, for example, see ref. 16 . Stalks are mainly composed of polysaccharides associated with poorly crystalline Fe(III) oxyhydroxides, however, the exact composition of their organic matrix is unknown [17] . Although mineralized twisted filaments are commonly described as ancient microaerophilic FeOB in the rock record or in hydrothermal deposits, for example, see refs 18 , 19 , 20 , it is unknown how the twisted stalk organic matrix and mineralogy evolve as a function of T and P conditions typical of diagenesis. Recently, Chan et al . [21] demonstrated that twisted stalks are biological structures formed during cell growth and Fe(II) oxidation [21] . Stalks have thus been proposed as morphological biosignatures for FeOB [18] , [21] . As stalk formation is induced by O 2 in cultures of Gallionella ferruginea [22] , and occurs at O 2 concentrations as low as 3 μM in cultures of Mariprofundus ferrooxydans [18] , stalks could also serve as evidence for the presence of localized oxygen in ancient environments. Here we study twisted stalks developing in a mat at an iron seepage in an abandoned mine. To evaluate how twisted stalks evolve when they get buried into sediments that will eventually become rocks, twisted stalks are submitted to T – P conditions typical of diagenesis. Using spectroscopy and microscopy, we characterize the changes in morphology, mineralogy and chemistry of the twisted stalks after incubations at up to 250 °C–140 MPa and for up to 16 weeks. We show that Fe minerals play a key role in maintaining the structural integrity of the twisted stalks and we infer that the association of organic polymers with Fe minerals helps preserving the twisted stalks under experimental diagenetic conditions. We provide morphological, mineralogical and spectroscopic signatures and their associated T – P conditions that could serve to clearly assign mineralized filaments to ancient activity of FeOB in diagenetically altered sediments. Fe(III) oxyhydroxides and stalk structural integrity A natural microbial mat was collected on the wall of an abandoned silver mine (Segen Gottes Mine, SW Germany; Fig. 1a ). Twisted stalks were the main components of the mat ( Fig. 1b ). Stalks were not attached to cells, most probably because cells break easily from the stalks during sample handling [21] , [23] . In scanning electron microscopy (SEM) images, stalks had a smooth surface with round aggregates ( Fig. 1c ), similarly to samples recovered in another underground environment [24] . Minerals in the original mat sample were X-ray amorphous or poorly crystalline as shown by a featureless X-ray diffractogram ( Supplementary Fig. 1 ). Raman spectroscopy identified the amorphous mineral phase in the original sample as ferrihydrite, a poorly ordered Fe(III) oxyhydroxide ( Fig. 2a ). In previous studies, poorly crystalline Fe(III) oxyhydroxides were identified at the surface of natural and cultured stalks, for example, see (refs 21 , 25 , 26 , 27 , 28 ). Akaganeite and lepidocrocite were also shown to occur on stalks, forming from the recrystallization of ferrihydrite [17] , [21] . It was suggested that haematite could form inside the fibres of the stalks as well [24] . 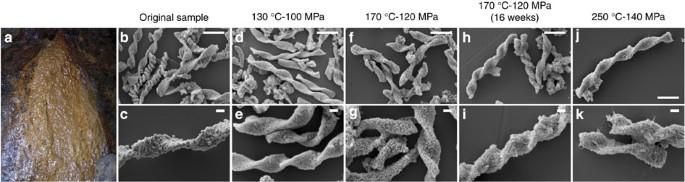Figure 1: Iron-oxidizing mat and twisted stalks as a function of pressure and temperature. (a) Fe(II)-oxidizing mat on a wall of the Segen Gottes Mine (SW Germany). (b–k) SEM images of twisted stalks before (original sample,b,c) and after incubations of 1 week at 130 °C–100 MPa (d,e), at 170 °C–120 MPa (f,g), and at 250 °C–140 MPa (j,k) and of 16 weeks at 170 °C–120 MPa (h,i). SEM images were obtained from Pt-coated samples, previously rinsed with water and air-dried. Scale bars are 5 μm (b,d,f,h,j) and 1 μm (c,e,g,i,k). Figure 1: Iron-oxidizing mat and twisted stalks as a function of pressure and temperature. ( a ) Fe(II)-oxidizing mat on a wall of the Segen Gottes Mine (SW Germany). ( b – k ) SEM images of twisted stalks before (original sample, b , c ) and after incubations of 1 week at 130 °C–100 MPa ( d , e ), at 170 °C–120 MPa ( f , g ), and at 250 °C–140 MPa ( j , k ) and of 16 weeks at 170 °C–120 MPa ( h , i ). SEM images were obtained from Pt-coated samples, previously rinsed with water and air-dried. Scale bars are 5 μm ( b , d , f , h , j ) and 1 μm ( c , e , g , i , k ). 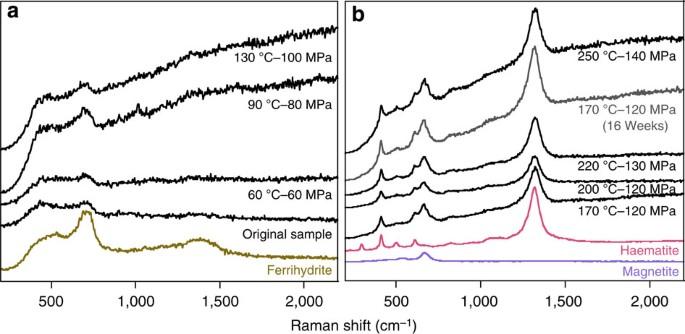Figure 2: Raman spectroscopic signatures of twisted stalks as a function ofTandPconditions. Raman spectra were acquired on bulk air-dried samples and on powders of the reference Fe minerals ferrihydrite, haematite and magnetite. Ferrihydrite coating the stalks was preserved at conditions including 130 °C–100 MPa (a) and transformed to haematite and magnetite at 170 °C–120 MPa (b). All conditions were applied for 1 week, unless otherwise stated. Full size image Figure 2: Raman spectroscopic signatures of twisted stalks as a function of T and P conditions. Raman spectra were acquired on bulk air-dried samples and on powders of the reference Fe minerals ferrihydrite, haematite and magnetite. Ferrihydrite coating the stalks was preserved at conditions including 130 °C–100 MPa ( a ) and transformed to haematite and magnetite at 170 °C–120 MPa ( b ). All conditions were applied for 1 week, unless otherwise stated. Full size image We observed the twisted stalks by SEM after a 0.5 N HCl treatment to dissolve ferrihydrite and ferric iron complexed by organic molecules ( Fig. 3 ). The organic stalk material almost completely disintegrated and lost its morphology when the sample was recovered by centrifugation after HCl treatment ( Fig. 3a ). When the sample was treated with HCl directly on the coverslip used for SEM (see sample preparation in the Methods section), we observed flat residues of stalks that were low in secondary electron contrast in SEM images ( Fig. 3b–e ), suggesting a crucial role for Fe(III) oxyhydroxides in maintaining the twisted stalk structural integrity at ambient conditions. 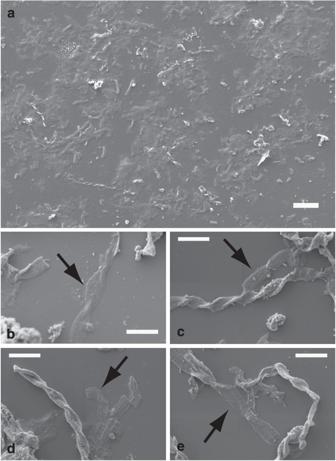Figure 3: SEM images of stalks treated with HCl 0.5 N. Either the sample was treated with HCl in a tube, then rinsed and centrifuged (a), or the sample was treated and rinsed directly on the coverslip that served as a support for SEM samples (b–e; see sample preparation in the Methods section). After complexed Fe(III) has been extracted and ferrihydrite has been dissolved, stalks lose their physical integrity, suggesting the importance of Fe(III) oxyhydroxides in maintaining the twisted structure. Arrows indicate flat stalks. Scale bars, 20 μm (a) and 5 μm (b,c,d,e). Figure 3: SEM images of stalks treated with HCl 0.5 N. Either the sample was treated with HCl in a tube, then rinsed and centrifuged ( a ), or the sample was treated and rinsed directly on the coverslip that served as a support for SEM samples ( b – e ; see sample preparation in the Methods section). After complexed Fe(III) has been extracted and ferrihydrite has been dissolved, stalks lose their physical integrity, suggesting the importance of Fe(III) oxyhydroxides in maintaining the twisted structure. Arrows indicate flat stalks. Scale bars, 20 μm ( a ) and 5 μm ( b , c , d , e ). Full size image Stalk morphology is preserved during experimental diagenesis Twisted stalks were submitted to T and P conditions typical of diagenesis—up to 250 °C and up to 140 MPa. Twisted stalks were clearly recognizable in SEM images after 1 week of incubation at all T – P conditions (130 °C–100 MPa, Fig.1d,e ; 170 °C–120 MPa, Fig. 1f,g , 250 °C–140 MPa, Fig. 1j,k ), and after a 16-week-long incubation at 170 °C–120 MPa ( Fig. 1h,i ). The average stalk length decreased significantly with increasing T – P conditions and with increasing time at 170 °C–120 MPa ( Fig. 4 , t -tests in Supplementary Table 1 ). The average stalk width did not vary significantly as a function of T – P conditions or as a function of time ( Fig. 4 , t -tests in Supplementary Table 2 ). The average widths in our study were between those of M. ferrooxydans stalks in cultures (1.1 μm±0.3 s.d.) and those of stalk microfossils in a hydrothermal deposit (3.9 μm±0.8 s.d.) [18] . 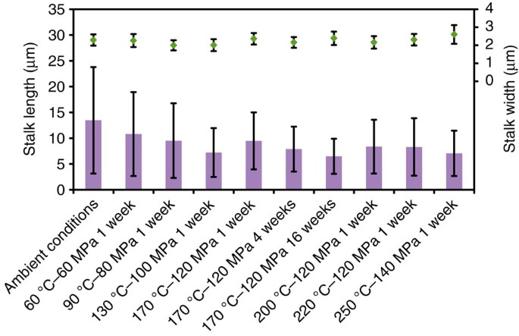Figure 4: Evolution of average stalk length and average stalk width as a function ofT–Pconditions and incubation time. The average stalk length (purple bars) decreased with increasingT–Pconditions, but also with incubation time (at 170 °C–120 MPa). The average stalk width (green diamonds) did not significantly vary as a function ofT–Pconditions or time. Error bars represent standard deviation of average stalk length and width. SeeSupplementary Fig. 2andSupplementary Tables 1and2for numbers of stalks measured for each condition and forPvalues oft-tests. Figure 4: Evolution of average stalk length and average stalk width as a function of T–P conditions and incubation time. The average stalk length (purple bars) decreased with increasing T–P conditions, but also with incubation time (at 170 °C–120 MPa). The average stalk width (green diamonds) did not significantly vary as a function of T–P conditions or time. Error bars represent standard deviation of average stalk length and width. See Supplementary Fig. 2 and Supplementary Tables 1 and 2 for numbers of stalks measured for each condition and for P values of t -tests. Full size image Changes in stalk mineralogical textures and composition Although the general twisted morphology of the stalks was not altered, the texture at the surface of stalks evolved from smooth and round aggregates at ambient conditions ( Fig. 1c ) to fine needles at 130 °C–100 MPa ( Fig. 1e ), to platelet-like structures at 170 °C–120 MPa ( Fig. 1g ) that were not altered within 4 months of incubation ( Fig. 1i ). The latter platelets started forming a network at the surface of the stalks at 250 °C–140 MPa ( Fig. 1k ). The textures observed in this study were unique to T – P conditions and, to our best knowledge, were never reported previously in natural mat samples or cultures. The twisted stalk surface alterations and the darkening of the mat colour from orange to dark red as T – P conditions increased pointed towards mineralogical and/or crystallinity changes. Up to 130 °C–100 MPa, ferrihydrite was the unique Fe phase ( Fig. 2a ), while it transformed into haematite and magnetite at 170 °C–120 MPa ( Fig. 2b and Supplementary Fig. 1 ). As no Fe(II) was present in the original sample, the formation of magnetite was attributed to Fe(III) reduction associated with organic matter oxidation as observed by Posth et al . [29] in a recent study. The signals of ferrihydrite in Raman spectroscopy and X-ray diffraction (XRD) being masked when crystalline phases are present, we cannot rule out the possibility that some fraction of ferrihydrite remained after incubation at high T – P conditions. As Raman spectroscopy and XRD are not quantitative techniques in these experimental conditions, we were not able to quantify the fractions of the different mineral phases in the samples after incubation. Twisted stalk organic matrix as a function of T and P The sample volume contained in gold capsules was limited to ~100 μl. After dissolution of Fe(III) oxyhydroxides, the remaining organic precipitate represented only a few % in volume. Therefore, bulk organic carbon analysis could not be performed. Moreover, acidic solutions used to dissolve the Fe(III) oxyhydroxides modify the composition of organic matter. Raman spectroscopy ( Fig. 2 ) did not yield any signal from carbon, for example, the broad G-band at ~1,600 cm −1 and D-band at ~1,350 cm −1 , due to the low content of organic carbon in the stalks. Therefore, for a detailed characterization and localization of the organic carbon before and after T – P treatment, we used spectroscopic and microscopic techniques that were compatible with small sample size and with the presence of large amounts of Fe minerals, namely scanning transmission X-ray microscopy (STXM) in combination with near edge X-ray absorption fine structure (NEXAFS) spectroscopy at the C1s edge at a 30-nm spatial resolution and confocal laser scanning microscopy (CLSM). NEXAFS spectra at the C1s edge recorded on single stalks at various T – P conditions ( Fig. 5a,b ) showed similar features to those reported for the stalk-producing FeOB M. ferrooxydans [21] , but different from those reported for stalk-producing FeOB from a mine [17] . Similar to the studies cited above, stalks from the Segen Gottes Mine did not contain inorganic C, as indicated by the absence of the C1s→π* excitation of the C=O bond in the carbonate at ~290.2 eV. In the stalk spectra, the shoulder at ~287.4 eV and the absorption peak at ~288.6 eV were characteristic of aliphatic and carboxylic carbons, respectively, suggesting the dominant presence and preservation of saturated lipids and polysaccharides in the stalks at all conditions ( Fig. 5a, b ). Organic carbon did not significantly change with increasing T – P conditions or experimental duration as indicated by the general shape of the NEXAFS spectra collected on the residues of each experiment ( Fig. 5a, b ). Carbon remained homogeneously distributed in the stalks at all conditions, as shown by the C1s average images ( Fig. 5c ). 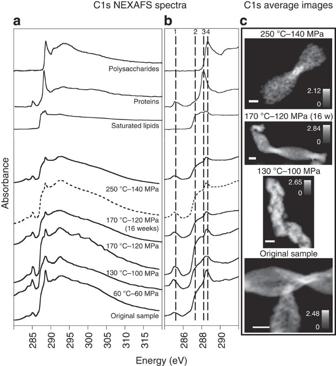Figure 5: Spectroscopic characterization by STXM-NEXAFS of biochemical compounds in twisted stalks as a function of T and P. All conditions were applied for 1 week, unless otherwise stated. (a) C1s NEXAFS spectra of reference compounds—saturated lipids (1,2 dipalmitoyl-sn-glycero-3-phosphocholine), polysaccharides (alginate) and proteins (albumin) and of twisted stalks before and after incubations at variousT–Pconditions. (b) C1s NEXAFS spectra fromarepresented over narrower range of energies. Dashed lines indicate energies at 285.5 (1), 287.4 (2), 288.2 (3) and 288.6 (4) eV interpreted as 1s→π* excitations of aromatic C (1), 1s→σ* excitations of aliphatic C (2), 1s→π* excitations of C=O next to the peptidic bond (3) and 1s→π* excitations of C=O in carboxylic C (4). (c) C1s average images (average optical density, 280–320 eV) in twisted stalks from the following samples: original sample, sample incubated at 130 °C–100 MPa for 1 week, sample incubated at 170 °C–120 MPa for 16 weeks and sample incubated at 250 °C–140 MPa for 1 week. Scale bars, 1 μm on all images. Figure 5: Spectroscopic characterization by STXM-NEXAFS of biochemical compounds in twisted stalks as a function of T and P. All conditions were applied for 1 week, unless otherwise stated. ( a ) C1s NEXAFS spectra of reference compounds—saturated lipids (1,2 dipalmitoyl-sn-glycero-3-phosphocholine), polysaccharides (alginate) and proteins (albumin) and of twisted stalks before and after incubations at various T–P conditions. ( b ) C1s NEXAFS spectra from a represented over narrower range of energies. Dashed lines indicate energies at 285.5 (1), 287.4 (2), 288.2 (3) and 288.6 (4) eV interpreted as 1s→π* excitations of aromatic C (1), 1s→σ* excitations of aliphatic C (2), 1s→π* excitations of C=O next to the peptidic bond (3) and 1s→π* excitations of C=O in carboxylic C (4). ( c ) C1s average images (average optical density, 280–320 eV) in twisted stalks from the following samples: original sample, sample incubated at 130 °C–100 MPa for 1 week, sample incubated at 170 °C–120 MPa for 16 weeks and sample incubated at 250 °C–140 MPa for 1 week. Scale bars, 1 μm on all images. Full size image The stalks did not bind the fluorescent dye Nile Red (specific for neutral lipids) while they did bind the lipophilic styryl dye FM4-64. Because of the limited amount of samples in the gold capsules, a characterization of lipids in the stalks is not possible. Similar to our study, Chan et al . [21] observed the presence of aliphatic C in their C1s NEXAFS measurements of M. ferrooxydans stalks. However, as the stalks did not bind the Nile Red dye, the authors concluded that stalks did not contain lipids [21] . Three different lectins could bind to the stalks: concanavalin A, specific to α-mannopyrosyl and a-glucopyrosyl residues; peanut agglutinin, specific to terminal β-galactose residues and wheat germ agglutinin, specific to N -acetyl-glucosamine and N -acetyl-neuraminic acid ( Supplementary Fig. 3 ). Lectins were heterogeneously bound to the stalks and the binding affinity remained heterogeneous at all T – P conditions ( Supplementary Figs 4 and 5 ). The protein-specific fluorescent dye NanoOrange did not bind the stalks. As shown in other studies, proteins are a minor component of the twisted stalks [21] , [30] , [31] . Spectroscopic signatures of the twisted stalk organic matrix We used μ-Fourier transform infrared (FTIR) spectroscopy measurements to characterize further the organic matrix ( Fig. 6 ). The presence of bands at 2,955–2,961, 2,921–2,927 and 2,852–2,854 cm −1 is characteristic of C–H stretching in CH 3 and CH 2 groups and indicative of aliphatic compounds ( Fig. 6 , bands 1, 2 and 3). The intensity of the stretching bands from CH 2 groups (bands 2 and 3) relative to the ones from CH 3 groups (band 1) suggests that aliphatic chains are linear or contain limited branching. The lack of a visible contribution from bands above 3,000 cm −1 , from the stretching vibrations of =C–H groups, also suggests that these aliphatic chains are mostly or fully saturated. The identification of individual molecules by FTIR spectroscopy is unfortunately not possible. However, from the spectral features described above, we can infer that these compounds are alkyl chains without functional groups, or alkyl chains with either hydroxyl groups (long-chain alcohols) or carboxyl groups (fatty acids). Unfortunately, we cannot discriminate further among these possibilities. If present, the functional groups carboxyl and/or hydroxyl would be limited in number in comparison to CH 3 and CH 2 groups, thus the intensity of their bands would be too weak to be distinguished. Given that the NEXAFS data indicated the presence of saturated lipids, the most plausible compounds are lipid compounds (for example, fatty acids). Although the peak intensities of bands 1, 2 and 3 decreased in the sample incubated for 1 week at 250 °C–140 MPa and for 16 weeks at 170 °C–120 MPa, the peaks were still present indicating the preservation of the lipid-like compounds under conditions of experimental diagenesis. The presence of lipids has been reported in sheaths produced by the FeOB Leptothrix [32] . Remains of lipids are known as the best-preserved biomarkers and have been recovered from ancient sediments [33] . Although we were not able to determine the exact lipid components, we provide a spectroscopic signature of organic carbon for microaerophilic FeOB in addition to the twisted stalk morphology. The μ-FTIR spectra also contained bands typical of polysaccharides in the region 800–1,200 cm −1 ( Fig. 6 , bands 5, 7, 8, 10, 11 and 12). However, their presence was not dependent on T – P conditions, suggesting that the polysaccharide composition changed from a stalk to another. As shown in the CLSM data ( Supplementary Figs 4 and 5 ), the heterogeneity of the polysaccharides was preserved as T – P conditions increased. A broad band at 1,048–1,058 cm −1 appeared on the IR absorption spectra at 170 °C–120 MPa and remained present at higher T – P conditions, covering a part of the range of interest for polysaccharides ( Fig. 6 , band 9). This band is most probably the signature of crystalline SiO 2 that formed at high T – P conditions from the little amount of Si present in the original sample (5 wt% as detected by SEM-energy-dispersive spectroscopy). 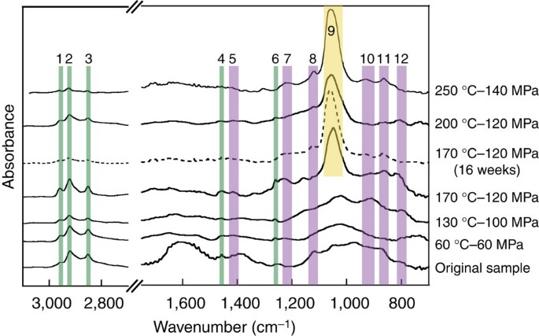Figure 6: FTIR fingerprints of twisted stalks as a function of pressure and temperature. Synchrotron μ-FTIR spectra were recorded on air-dried single stalks. All conditions were applied for 1 week, unless otherwise stated. Bands 1, 2, 3, 4, 6 are the fingerprints of vibrations of CH2(2,921–2,927 and 2,852–2,854 cm−1) and CH3(2,955–2,961, 1,450 and 1,260 cm−1) in aliphatic chains and are preserved at allT–Pconditions tested. Bands 5, 7, 8, 10, 11, 12 are the fingerprints of polysaccharides (1,415, 1,250, 1,120, 910–930, 860 and 805 cm−1). They appear independently of theT–Pconditions suggesting the heterogeneity of the polysaccharide distribution, as confirmed by the CLSM data (Supplementary Figs 4and5). Band 9 is the fingerprint of silicate minerals. Bands typical of proteins (amide I and amide II) are not visible on the spectra, certainly due to the low amount of proteins in the twisted stalks. Figure 6: FTIR fingerprints of twisted stalks as a function of pressure and temperature. Synchrotron μ-FTIR spectra were recorded on air-dried single stalks. All conditions were applied for 1 week, unless otherwise stated. Bands 1, 2, 3, 4, 6 are the fingerprints of vibrations of CH 2 (2,921–2,927 and 2,852–2,854 cm −1 ) and CH 3 (2,955–2,961, 1,450 and 1,260 cm −1 ) in aliphatic chains and are preserved at all T–P conditions tested. Bands 5, 7, 8, 10, 11, 12 are the fingerprints of polysaccharides (1,415, 1,250, 1,120, 910–930, 860 and 805 cm −1 ). They appear independently of the T – P conditions suggesting the heterogeneity of the polysaccharide distribution, as confirmed by the CLSM data ( Supplementary Figs 4 and 5 ). Band 9 is the fingerprint of silicate minerals. Bands typical of proteins (amide I and amide II) are not visible on the spectra, certainly due to the low amount of proteins in the twisted stalks. Full size image The structural integrity of the twisted stalks appears maintained by Fe phases ( Fig. 3 ), similar to the shape of microbial cells preserved by Fe 3+ during fossilization experiments at ambient conditions. The cell wall structure of the archaeon Methanocaldococcus janaschii was preserved in silica only when cells have been in contact with Fe 3+ (ref. 8 ). Preservation of the cell wall of the bacterium Bacillus subtilis was greatly enhanced after cells bound Fe 3+ , which inhibited autocatalytic enzymes [9] . However, after incubation at 100 °C, Fe 3+ cations bound to the cell wall did not maintain B. subtilis cell shape and cell wall structure [34] . The shape of Acidovorax sp. BoFeN1 cells, when encrusted in Fe(III) oxyhydroxides, is preserved after 100 h at 300 °C and after 20 h at 600 °C (ref. 12 ). We thus infer that cells or extracellular structures associated to Fe minerals are more likely to be preserved under diagenetic conditions than those bound to Fe 3+ . As Fe phases become more crystalline and stable between 130 °C–100 MPa and 170 °C–120 MPa, they have the potential to preserve stalk morphology over long periods of time under diagenetic conditions. We document the preservation of both main components of the twisted stalk organic matrix—long-chain saturated aliphatic compounds and polysaccharides—under diagenetic conditions ( Figs 5 and 6 ). Previous studies detected acidic polysaccharides, similar to alginate, as the dominant component of the organic matrix in twisted stalks produced by the marine FeOB M. ferrooxydans [21] , in twisted stalks of the freshwater FeOB Sideroxydans R-1 31 and in stalks collected in a mine [17] . As Fe potentially binds to carboxylic groups of the organic polymers [21] , the role of iron in the diagenesis of organic matter becomes a central question. In modern aquatic sediments, more than 20% of the labile organic matter is stabilized by the formation of complexes between organic matter and reactive iron that are not accessible for microbial degradation [35] . At deep-sea hydrothermal vents, Fe(II) and organic matter form complexes, preserving both components after hydrothermal fluids have been in contact with oxygenated seawater [36] . As diagenetic conditions occur, organic matter could also protect amorphous Fe phases from further modifications. The temperature at which ferrihydrite transforms into crystalline phases is dependent on the association of ferrihydrite with organic matter, but also on the amount and quality of organic matter associated with it [29] , [37] , [38] . Kennedy et al . showed that pure ferrihydrite transformed to haematite at 80 °C, whereas it remained stable when associated with bacteria at the same temperature [38] . Using experimental conditions similar to ours, Posth et al . [29] demonstrated that, after 14 days at 170 °C–120 MPa, ferrihydrite alone transformed to haematite while ferrihydrite associated with glucose completely transformed to haematite, magnetite and siderite [29] . Interestingly, biogenic ferrihydrite recovered at deep-sea hydrothermal vents was preserved after heating 20 min up to 400 °C and transformed to haematite only at 500 °C (ref. 37 ). Here we provide the T – P conditions at which mineralogical transformations specifically occur in twisted stalks. We propose that the Fe minerals, as they transform to crystalline and stable phases, act as a physical protection for the organic matrix and help preserving the main organic components under diagenetic conditions. We show that Fe-mineralized stalks are extremely resistant under experimental diagenetic conditions for up to 16 weeks ( Figs 1 , 5 and 6 ). We can simulate the T – P conditions of diagenesis in the laboratory, yet it remains a challenge to extrapolate the fate of the twisted stalks to geological durations. We show that the length of the stalks decrease with increasing T – P conditions, as well as with time at 170 °C–120 MPa ( Fig. 4 and Supplementary Fig. 2 ). Therefore, it is possible that stalks be eventually destroyed after long periods of time at these T – P conditions. In a study of the filamentous cyanobacterium Lyngbya majuscule under diagenetic conditions, sheaths and cells showed only slight structural alteration after a 31-week incubation at 100 °C–300 MPa (refs 14 , 15 ). However, after 2 weeks at 165 °C–300 MPa, sheaths broke and cell size was significantly reduced, whereas after 3–4 weeks sheaths were highly degraded and cells hardly visible [14] , [15] . In natural environments, stalks accumulate various amounts of Fe minerals and can appear heavily encrusted [39] . Therefore, it is possible that crystal growth continues if diagenetic conditions are maintained for long durations and that stalk morphology and mineral textures become completely obliterated. Finally, we show that magnetite forms in the stalks at high T – P conditions, suggesting that some organic carbon oxidation occurs with Fe(III) reduction at high temperature and/or pressure. Organic compounds in microbial cells undergo modifications under various conditions of T and P , as shown in the following studies. The evolution of the organic matter in cultures of Methanocaldococcus jannashii was investigated during a 1-year silicification experiment at 60 °C (ref. 40 ). Although cells were completely degraded after a year, the amount and composition of amino acids and fatty acids did not significantly changed. The most abundant sugar glucose was still detected after a year, whereas mannose, a less abundant sugar, completely disappeared [40] . Bacteriohopanepolyols—lipid compounds found in bacterial membranes—of the purple non-sulfur bacterium Rhodopseudomonas palustris strain TIE-1 undergo modifications under diagenetic conditions similar to the ones used in our study [41] . Finally, the organic content of Fe-encrusted Acidovorax sp. BoFeN1 cells is modified after 100 h at 300 °C and after 20 h at 600 °C, with a significant decrease in the protein amount [12] . In addition, Fe minerals have been shown to promote catalytic decarboxylation of fatty acids in vitro at diagenetic temperatures [42] . Although the composition of the organic matter of stalks is different from cells, we can infer that both main components of the stalks—lipids and polysaccharides—will undergo further oxidation with time, leaving a twisted structure, if preserved, devoid of organic signatures that could eventually be filled by other minerals. Microaerophilic FeOB have been implicated in the oxidation of Fe(II), and deposition of oxidized Fe to iron formations (IF) [43] , [44] . Filaments or stalks coated with Fe oxyhydroxides have been reported in chert layers of the 1.89 Ga Gunflint IF [3] , [19] , [45] , in the 1.88 Ga Frere IF [46] , in the 1.88 Ga Sokoman IF [47] , in the 1.8 Ga Duck Creek IF [48] , [49] , and in the 1.7 Ga IF of the Jerome District, AZ [50] . The absence of twisted stalks in IF older than 1.89 Ga has been proposed as evidence that stalk-forming communities did not exist at that time [19] , [51] . Our work demonstrates that morphological, mineralogical and spectroscopic organic signatures associated with twisted stalks can be preserved under T – P conditions characteristic of the best-preserved late Archean IF of Western Australia or South Africa [52] , at least at the laboratory timescale. As twisted stalks can form at O 2 concentrations as low as 3 μM (ref. 18 ), microaerophilic FeOB might have been present before 1.9 Ga, but twisted stalks older than that age might as well have been degraded enough to be undetectable in the rock record. For example, microbial Fe(III) reduction, which is an ancient microbial process occurring readily in subsurface environments at the temperature limits for life, might have played a role [53] . So far it is unknown if the organic matrix of the stalks could serve as carbon source for Fe(III) reducers. Our results underline the importance of microbial extracellular structures for the search of ancient life in deposits having experienced a diagenetic history. Cyanobacterial sheaths are generally more resistant than cells under diagenetic conditions [14] , [15] . As stalk-forming microorganisms avoid cell encrustation by direct deposition of Fe(III) oxyhydroxides to the stalks [21] , Fe-free cells are thus likely to disappear under diagenetic conditions. Other microaerophilic FeOB produce mineralized extracellular appendages, such as sheaths or filaments. So far the evolution of these structures has not been investigated under diagenetic conditions. The importance of FeOB in marine environments has been recently recognized. The twisted stalk morphology has been observed in mats or precipitates at deep-sea hydrothermal environments such as seamounts [54] or spreading centres [55] , [56] , [57] and in shallow hydrothermal ferruginous sediments [58] , [59] . Although the twisted stalks are formed at relatively low temperatures, our results show that they will be potentially preserved even if T – P conditions change over time, for example, because of a change in the local hydrothermal regime. Assuming an ancient FeOB mat formed at 5,000 m water depth near a low-temperature hydrothermal system and subsequently buried in sediments, twisted stalks from that mat could actually be preserved up to 8 km below the seawater–sediment interface. Although organo-mineral twisted stalks, as used in our study, are rather unique to microbial microaerophilic Fe(II) oxidation [21] , twisted structures might be produced under abiotic conditions [60] . We thus propose that if structures similar to twisted structures are found in natural, lithified sediments, these should be characterized using spectroscopy using our criteria for an FeOB origin, in combination with those of Krepski et al . [18] for determining environmental conditions. Environmental samples and experimental diagenesis The source of the samples for the diagenesis experiments was an Fe(II)-oxidizing microbial mat growing on a tunnel wall of the ancient silver mine Segen Gottes in Haslach-Schnellingen (Black Forest, SW Germany). The microbial mat was sampled twice (November 2011 and March 2012) using sterile syringes. Samples were stored at 4 °C until used for diagenesis experiments in a high T and high P autoclave that functioned with water as pressure-transmitting medium (SITEC 01603-1500-R300 °C, SITEC-Sieber Engineering AG, Switzerland). Samples were incubated in gold capsules prepared from gold tubes (inner diameter 2.1 mm, outer diameter 2.5 mm, Wieland Edelmetalle GmbH, Pforzheim, Germany) combusted at 800 °C for 4 h. Capsules were sealed at one extremity by tungsten inert gas welding, sonicated in ethanol and dried at 60 °C before filling. Capsules were filled with ~100 μl of aqueous thick mat using sterile needles and syringes. The second extremity of the capsules was clamped and welded. After incubation, capsules were opened with a clean razor blade and samples were recovered using sterile micropipettes. Samples were 1/air-dried with or without a previous wash with sterile distilled water and air-dried or 2/used wet, depending on the measurements performed (see below). Geochemistry The total iron content of a dissolved mat sample (70 °C in 6 N HCl, 48 h) was 0.99 g l −1 as measured by ferrozine assay. No Fe(II) was present in the mat sample. The pore water was extracted by centrifugation, filtered with a 0.22-μm cellulose filter, acidified with HNO 3 and analysed using inductively coupled plasma atomic emission spectroscopy ICP-OES and inductively coupled plasma mass spectrometry (ICP-MS). The following metals were measured: As (47.3 μg l −1 ), B (37.2 μg l −1 ), Co (9.3 μg l −1 ), Cr (1.3 μg l −1 ), Cu (1.8 μg l −1 ), Fe (59.0 μg l −1 ), Ni (21.5 μg l −1 ), Zn (6.49 mg l −1 ) and Mn (1.05 mg l −1 ). Scanning electron microscopy SEM analyses were performed with a LEO 1450 VPSEM equipped with a tungsten hairpin filament (now Zeiss) at the Department of Geosciences (University of Tübingen). A drop of sample washed in sterile distilled water was deposited and air-dried on a circular glass coverslip that was attached to an aluminium stub with double-side carbon tape. Samples were sputter-coated with ~8 nm of Pt with a BalTec SCD 005 sputter coater (BalTec, Liechtenstein). Images were acquired with an acceleration voltage of 5 kV and at a working distance of 3–4 mm using an Everhart-Thornley secondary electron detector. Raman spectroscopy Raman spectra were measured using an Alpha300 Raman spectrometer (WITec) at the Department of Pharmaceutical Technology (University of Tübingen). The spectrometer was equipped with CCD and 1,800 grooves per mm grating. The excitation source was a 534-nm-line laser with power of light evaluated at <1 mW on the sample. Each Raman spectrum was an average of two accumulations of 60 s. Measurements were done on air-dried samples deposited on a glass slide. Synthetic Fe oxyhydroxides were used as reference compounds and measured as dry powders on a glass slide. Goethite, magnetite (Bayferrox, LANXESS Inorganic Pigments) and haematite (Fluka >99%) were purchased, whereas ferrihydrite was synthesized in the laboratory using a standard protocol [61] . Micro-X-ray diffraction (μ-XRD) μ-XRD data were collected with a Bruker D8 Discovery XRD instrument (Bruker) equipped with a Co-Kα X-ray tube ( λ =0.17902, nm, 30 keV, 30 mA) and GADDS area detector [62] . Samples were air-dried and mounted on a Si single-crystal silicon wafer. Confocal laser scanning microscopy CLSM measurements were performed on a Leica SPE confocal laser scanning microscope (Leica Microsystems) equipped with 405, 488, 561 and 635 nm lasers and a × 63 water immersion lens with a numerical aperture of 1.15 at the Center for Applied Geoscience (Environmental and Analytical Microscopy group, University of Tübingen). The following fluorescent probes (Molecular Probes, Life Technologies) were tested on the samples—the stain NanoOrange for proteins, various lectin-Alexa Fluor conjugates of peanut agglutinin, concanavalin A and wheat germ agglutinin for polysaccharides and the stains FM4-64 and Nile Red for lipids. STXM and NEXAFS spectroscopy STXM and NEXAFS spectroscopy measurements were performed at the spectromicroscopy beamline 10ID1 of the Canadian Light Source (CLS, Saskatoon, SK) [63] . The STXM instrument uses a Fresnel zone plate to focus the X-ray to a spot size of 30 nm. The beamline, equipped with a plane grating monochromator was operated at an energy resolution of <0.1 eV at the C1s absorption edge. Image sequences (stacks) were recorded on single stalks across the C1s edge (280–320 eV) with energy steps of 0.29 eV (280–284.2 eV), 0.1 eV (284.2–291.9 eV), 0.3 eV (291.9–300 eV) and 0.6 eV (300–320 eV) and a dwell time of 1 ms per pixel. The native mat sample and the samples recovered from the capsules after T – P incubations were rinsed and re-suspended in filtered distilled water. A drop of suspension was deposited and air-dried on formvar-coated 200-mesh TEM (transmission electron microscopy) grids. Before measuring all samples under oxic conditions, STXM measurements were performed on a sample prepared under anoxic conditions (opened, rinsed with anoxic water, sandwiched between two silicon nitride windows sealed together with epoxy; all procedures performed in an anoxic glovebox). As no differences in Fe-redox states and organic speciation were observed between the two sample preparations, samples were further prepared on TEM grids. Data processing was performed using the aXis2000 software package [64] . Images were converted from transmission scale to linear absorbance scale (optical density, OD), using the equation: OD=−ln(I/I 0 ), where OD is the optical density of an individual pixel, I is the intensity of the transmitted photons and I 0 is the intensity measured in an empty area adjacent to the sample. NEXAFS spectra from stalks were extracted from image sequences collected across the C1s absorption edge. C1s average images (optical density) were generated by averaging all images recorded at energies between 280 and 320 eV. The reference spectra used in this study were NEXAFS C1s spectra of standard compounds alginate (used as polysaccharide standard), albumin (used as protein standard) and 1,2-dipalmotoyl-sn-glycero-3-phosphocholine (used as aliphatic compound standard). These compounds were shown to represent the major constituents of microbial biofilms in various studies [65] , [66] , [67] , [68] . Synchrotron infrared spectroscopy FTIR spectromicroscopy experiments were performed on Beamline X01DC of the Swiss Light Source (SLS). Samples were rinsed and diluted in sterile distilled water and air-dried on formvar-coated 200-mesh TEM grids. Samples were measured in the transmission configuration using a × 36 Schwarzschild objective/condenser pair. The instrument was setup for measurements in the mid infrared region by using a KBr-supported Ge-multilayer beamsplitter and a MCT detector. Acquisition was performed in double-sided, forward-backward mode, with a resolution of 4 cm −1 . Interferograms were phase-corrected with the Mertz algorithm, apodized with a Blackman-Harris three-term function and extended with a zero-filling factor of two before Fourier Transform. Measurements were performed in confocal geometry with the outgoing aperture set at 7 × 9 μm 2 . Four thousand scans were collected for each background and sample measurement. How to cite this article: Picard, A. et al . Experimental diagenesis of organo-mineral structures formed by microaerophilic Fe(II)-oxidizing bacteria. Nat. Commun. 6:6277 doi: 10.1038/ncomms7277 (2015).